Grain rotation mediated by grain boundary dislocations in nanocrystalline platinum Grain rotation is a well-known phenomenon during high (homologous) temperature deformation and recrystallization of polycrystalline materials. In recent years, grain rotation has also been proposed as a plasticity mechanism at low temperatures (for example, room temperature for metals), especially for nanocrystalline grains with diameter d less than ~15 nm. Here, in tensile-loaded Pt thin films under a high-resolution transmission electron microscope, we show that the plasticity mechanism transitions from cross-grain dislocation glide in larger grains ( d >6 nm) to a mode of coordinated rotation of multiple grains for grains with d <6 nm. The mechanism underlying the grain rotation is dislocation climb at the grain boundary, rather than grain boundary sliding or diffusional creep. Our atomic-scale images demonstrate directly that the evolution of the misorientation angle between neighbouring grains can be quantitatively accounted for by the change of the Frank–Bilby dislocation content in the grain boundary. Grain rotation is a well-known phenomenon for polycrystalline materials during deformation at high (homologous) temperatures [1] , [2] , [3] , [4] , [5] , [6] , [7] , [8] . It is also common during annealing and recrystallization in polycrystalline materials [9] , [10] , [11] . The proposed mechanisms mediating grain rotation include intra-grain dislocation processes (that is, the cross-grain glide of a large number of dislocations that re-orient the grains with respect to surrounding grains [2] ), diffusive mechanisms [3] , [4] as well as sliding [5] , [6] , [7] , [8] at the grain boundaries (GBs). In recent years, grain rotation has also been proposed as a plasticity phenomenon at low temperatures (for example, room temperature for metals), especially for nanocrystalline (NC) grains with a very small diameter ( d ) [12] , [13] , [14] , [15] , [16] , [17] , [18] , [19] , [20] , [21] . In the latter case, however, the underlying mechanism remains unclear: the glide of cross-grain dislocations is expected to subside in such tiny grains [12] , [13] , [14] , [15] , [22] , [23] , [24] , [25] , [26] , [27] , [28] , [29] , [30] , [31] , [32] , [33] , and diffusional processes may also be insufficient to mediate fast GB sliding at room temperature. Then how can grain rotation be realized to carry plasticity in such an NC system? The classical theories developed in the 1950’s and later [9] , [34] , [35] , [36] , [37] stipulate that such low-temperature grain rotation (that is, change of the misorientation angle between grains but not the apparent grain size) can be accomplished primarily by GB dislocations. However, so far there has been no direct and quantitative experimental evidence to verify that this is indeed the case. Here, by using a newly developed deformation device in a high-resolution transmission electron microscope (HRTEM), the atomic-scale and dynamic deformation process of NC Pt has been recorded in situ . We show direct and quantitative evidence that when the grain size is below ~6 nm, the plastic deformation mode becomes grain rotation, involving multiple grains in a collective manner. This particular process is mediated by the climb of GB dislocations, rather than cross-grain dislocation slip or GB sliding. In situ deformation of Pt NC thin film As shown in the bright-field TEM image of Fig. 1a , the Pt film has nanometre-sized and equi-axed grains, with no obvious texture (see the selected area diffraction patterns in the inset and Supplementary Fig. 1 ). The HRTEM image in Fig. 1b shows that most grains are separated by high-angle GBs, without visible porosity or micro-cracks. The cross-sectional TEM images indicate that the thin film is ~10 nm in thickness, and consists of one or two grains in the thickness direction ( Fig. 1c ). The distribution of grain sizes, as measured for ~180 grains, is shown in Fig. 1d . The grain diameters range from 2 to 12 nm and most of the grains have a diameter below 10 nm, with an average d of ~6 nm. Tensile experiments were carried out using our TEM tensile stage as shown in the schematic in Fig. 1e . This special stage allows slow and gentle deformation of the electron-transparent film, and at the same time retains the double-tilt capability such that the grains can be oriented appropriately to a low-index crystallographic zone orientation for high-resolution imaging (see refs 28 , 29 for details). The tensile pulling was realized by heating the sample holder to ~80 °C, causing bending of the bimetallic strips due to thermal expansion. The real-time evolution of the film was captured in situ along with deformation, in a JEOL-2010 field-emission TEM operating at 200 kV. 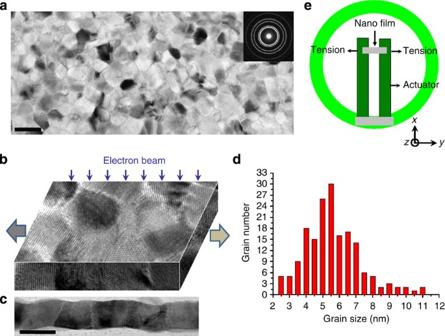Figure 1: TEM observations of the Pt nanocrystalline thin film. (a) Bright-field transmission electron microscope (TEM) image of the Pt film, with a selected area diffraction pattern in the inset. (b) High-resolution TEM (HRTEM) image showing grains separated by high-angle grain boundaries (GBs). (c) Cross-sectional TEM image of the thin film. (d) Statistical distribution of the grain size. (e) Home-made testing device used forin situtensile pulling of the Pt thin film in a TEM. Scale bars, 10 nm. Figure 1: TEM observations of the Pt nanocrystalline thin film. ( a ) Bright-field transmission electron microscope (TEM) image of the Pt film, with a selected area diffraction pattern in the inset. ( b ) High-resolution TEM (HRTEM) image showing grains separated by high-angle grain boundaries (GBs). ( c ) Cross-sectional TEM image of the thin film. ( d ) Statistical distribution of the grain size. ( e ) Home-made testing device used for in situ tensile pulling of the Pt thin film in a TEM. Scale bars, 10 nm. 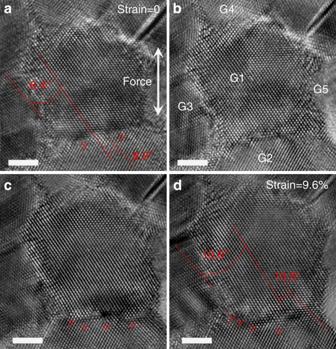Figure 2: HRTEM images taken at different points of time showing the GB dislocation-mediated grain rotation. (a) Two GB dislocations (as marked with ‘T’) at GB1–3. (b–d) During straining, the number of the dislocations increased, leading to the GB angle atG1–2increasing from 8.3° to 13.5°. Scale bars, 2 nm. Full size image Atomic-scale in situ observation of grain rotation in small grains Figure 2 is a series of HRTEM images, showing the GB dislocation-mediated grain rotation process observed at the atomic scale. For convenience, we define the in-plane motion about the axis parallel to the electron beam as ‘rotation’ and the out-of-plane rotation around an axis in the film plane as ‘tilt’. We define G i–j as the GB between grains G i and G j . As shown in Fig. 2a , both G 1 and G 2 exhibit a clear [110] (axis) lattice and the GB angles are 8.3° and 6.4° for G 1–2 and G 1–3 , respectively. In the figure, the double-ended arrow indicates the loading axis, relative to the grains G 1 , G 2 and G 3 . As revealed in Fig. 2b–d , during the straining, the number of the dislocations at G 1–2 increases and the average spacing of the GB dislocations decreases from 3.1 to 1.2 nm. This increased number of GB dislocations leads to the increased misorientation angle of G 1–2 , from 8.3° to 13.5°, as well as that of G 1–3, from 6.4° to 10.6°. No dislocations were observed inside the small grains throughout the deformation process. During the straining, G 1 and G 2 exhibit no obvious lattice fringe change, indicating that the grain rotation is not caused by a global tilt of specimen during deformation. Figure 2: HRTEM images taken at different points of time showing the GB dislocation-mediated grain rotation. ( a ) Two GB dislocations (as marked with ‘T’) at GB 1–3 . ( b – d ) During straining, the number of the dislocations increased, leading to the GB angle at G 1–2 increasing from 8.3° to 13.5°. Scale bars, 2 nm. Full size image As the grain size decreases, the grain rotation is more obvious. 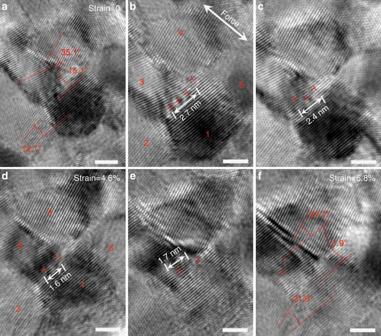Figure 3: Atomic-scalein situobservation of grain rotation in smaller grains. (a) An array of dislocations (as marked with ‘T’) forms a wedge-shaped disclination at the GB. (b–e) During straining, the number of the dislocations decreases, leading to decreasing GB angleG1–3. (e,f) The dislocation number decreases, caused by the GB dislocations climbing into the TJs or other GBs. Meanwhile, the GB angle atG1–2increased from 12.1° to 21.6°. Scale bars, 2 nm. Figure 3 is a series of HRTEM images, showing the GB dislocation-mediated grain rotation process at the atomic scale. Figure 3a highlights five grains ( d ~5 nm, marked as ‘1’ to ‘5’), separated by high-angle GBs. During the straining, G 3 and G 4 exhibit no obvious fringe change, indicating that there is no global tilt and shift of the specimen during deformation. The double-ended arrow in Fig. 3b indicates the loading axis. The GB angles are 12.1°, 15.1° and 35.1° for G 1–2 , G 1–3 and G 3–4 , respectively. As noted with ‘T’ in Fig. 3a , an array of GB dislocations can be seen at G 1–3 . As shown in Fig. 3b–f , during the in situ straining, the number of the dislocations at G 1–3 decreases and the average spacing of the GB dislocations increases from 0.9 to 1.7 nm. This corresponds to a reduced misorientation angle at G 1–3 , decreasing from 15.1° to 1.9°. Figre. 3e,h show that the GB dislocations have climbed towards the triple junction (TJ) points, and the dislocation annihilation/absorption in the TJ (or other GBs) is the reason of the decrease in the number of GB dislocations. For G 1–3 , the GB angle increased from 12.1° to 21.6°, while that for the G 3–4 decreased from 35.1° to 27.7°. Here again, no intra-grain dislocations were observed inside these tiny grains throughout the deformation process. It is noted that G 1 rotates about 9.5° with respect to G 2 but 13.2° with respect to G 3 . If only G 1 underwent the rotation process, the rotation angle of G 1 with respect to others would be the same. We also measured the rotation angles of G 1–4 , G 2–4 and G 2–3 . The rotation angles all exhibited different values. This indicates that these grains underwent a simultaneous rotation process, that is, they all participated in rotations relative to one another in a coordinated manner during straining. A number of in situ observations consistently show that for those grains surrounded by small grains, they underwent collective rotation together ( Supplementary Tables 1 and 2 , and Supplementary Fig. 2 ). For the grains surrounded by large grains, only the smaller grains underwent rotation (see next paragraph, Supplementary Table 3 and Supplementary Figs 3 and 4 ). Figure 3: Atomic-scale in situ observation of grain rotation in smaller grains. ( a ) An array of dislocations (as marked with ‘T’) forms a wedge-shaped disclination at the GB. ( b – e ) During straining, the number of the dislocations decreases, leading to decreasing GB angle G 1–3 . ( e , f ) The dislocation number decreases, caused by the GB dislocations climbing into the TJs or other GBs. Meanwhile, the GB angle at G 1–2 increased from 12.1° to 21.6°. Scale bars, 2 nm. 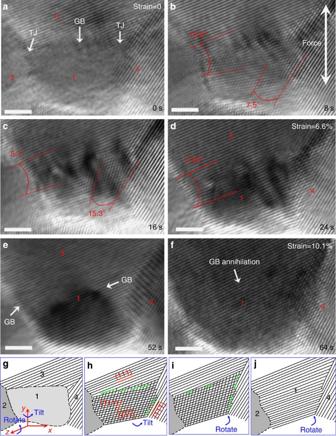Figure 4:In situobservation of the grain rotation for a 4.8 nm × 6.8 nm sized grain. The white arrow inbindicates the loading axis. Ina,G1is surrounded by high-angle GBs. (b,c) With straining,G1exhibits the [110] lattice, and the GBG1–3andG1–4have changed into small-angle GBs. (d,e) With further straining, the [110] axial-lattice inG1changed into fringes. (f) The GBG1–2disappeared andG1–4extended to become a long GB. (g–j) Schematics corresponding toa–fto illustrate the rotation process ofG1under tensile stress. Scale bars, 2 nm. Full size image Figure 4 presents a series of HRTEM images, showing another scenario for the rotation of a small grain, which underwent not only rotation but also tilt. As described above, the small grain G 1 ( d =4.8 nm) clearly exhibits GB dislocation-mediated grain rotation. In a larger grain, G 4 ( d >10 nm), full dislocations were frequently observed [28] , [29] , in lieu of grain rotation. During straining, no change was observed for the lattice/fringe in grains G 3 and G 4 ( Supplementary Figs 3 and 4 ), indicating that there was no rotation/tilt between G 3 and G 4 . In comparison, the contrast of the G 1 grain, and the GB structure of G 1–3 and G 1–4 , changed quickly. From Fig. 4a , G 1 is surrounded by high-angle GBs: no fringes were observed in G 1 , while G 3 and G 4 exhibit obvious fringes. The TJs are indicated by arrows. With increasing straining, we observed a clear [110] (axis) lattice ( Fig. 4b ) in G 1 , and the GB angles are 12.6° and 7.5° for G 1–3 and G 1–4 (they changed into small-angle GBs), respectively. This is obviously caused by the tilting of G 1 , together with GB structural changes. On further loading, the lattice in G 1 changed into fringes and then became the same as the grain G 3 ( Fig. 4c–f ), involving both in-plane and out-of-plane grain re-orientation. The G 1–3 changed from a high-angle GB to a small-angle GB and then disappeared, and the TJ changed into a GB. For G 1–4 , it changed from a small-angle GB (7.5° in Fig. 4b ) to a high-angle GB (15.3° in Fig. 4c ). Although the angle of G 1–3 cannot be measured after Fig. 4c , it continued to increase because of the rotation and tilt of the grain G 1 . In Fig. 4d,e , G 1–4 shows the features of a typical high-angle GB. Figure 4g–j presents the schematic view corresponding to Fig. 4a–f , for illustrating the rotation process of G 1 . As illustrated in Fig. 4g,h , the rotation and tilting of G 1 led to the appearance of lattice fringe in the image. The G 1–3 and G 1–4 consist of arrays of GB dislocations (as marked in green lines). With extensive deformation, G 1 rotated via GB dislocation motion and annihilation. The GB angles decreased (or increased) as the dislocation number changed, as shown in Fig. 4h,i . The continued rotation and tilting of G 1 eventually led to the merge of the grain as the GB in between and the TJ disappear ( Fig. 4j ). Here, G 1 was surrounded by relatively large grains (such as G 2 , G 3 and G 4 ). We can see that the rotation angle of G 1 with respect to G 3 and G 4 is the same, while the rotation angle of G 3 with respect to G 4 is nearly zero. Thus, only G 1 underwent the rotation process during deformation ( Supplementary Table 3 ). Figure 4: In situ observation of the grain rotation for a 4.8 nm × 6.8 nm sized grain. The white arrow in b indicates the loading axis. In a , G 1 is surrounded by high-angle GBs. ( b , c ) With straining, G 1 exhibits the [110] lattice, and the GB G 1–3 and G 1–4 have changed into small-angle GBs. ( d , e ) With further straining, the [110] axial-lattice in G 1 changed into fringes. ( f ) The GB G 1–2 disappeared and G 1–4 extended to become a long GB. ( g – j ) Schematics corresponding to a – f to illustrate the rotation process of G 1 under tensile stress. Scale bars, 2 nm. Full size image We also used black lines drawn on the {111} planes in grains G 1 , G 3 and G 4 to reveal the details of the GB dislocation-mediated grain rotation. These dark lines were derived from the actual atomic positions visible in HRTEM images to indicate an array of dislocations at G 1–3 . During straining, the number of dislocations at G 1–3 decreased along with the increased average spacing of the GB dislocations. This gradually decreased the GB angle of G 1–3 until its final annihilation ( Supplementary Fig. 5a–c,f–h ). For G 1–4 , the number of dislocations in the GB increased, leading to an increasing GB angle ( Supplementary Fig. 5d,e,i,j ). During the rotation process, the GB dislocations adjusted their spacing by climbing along the GBs concurrently, with increasing/decreasing number of GB dislocations. Meanwhile, the GB angle continuously changed. The dislocations climbed short distances to GB TJs and free surfaces, with no obvious cross-grain dislocation glide. Grain rotation and Frank–Bilby equation Clearly, the low-temperature grain rotation is not mediated by cross-grain glide of a large number of dislocations that re-orient the grain with respect to the surrounding grains [35] , [38] , [39] , nor diffusional creep processes [12] , [13] , [14] , [15] , [17] and GB sliding [17] , [18] . Instead, the grain rotation is found to be accomplished primarily by the change in the content of GB dislocations [34] , [35] , [36] , [37] . Such an evolution of GB dislocations is expected to cause a change in the GB angle between neighbouring grains, as indicated by the well-known Frank–Bilby equation [36] , [37] : Here we choose a proper vector p (lying in the GB) such that the Burgers circuit encloses all the GB dislocations. B is the sum of the Burgers vectors of the GB dislocations, θ is the GB angle and ρ is the rotation axis ( |ρ| ). According to equation (1), an increase in the number of GB dislocations would lead to increased B , and consequently increased GB angle θ . Conversely, decreasing the number of GB dislocations would reduce B and hence θ . This picture is exactly what we observe under the Cs-corrected HRTEM (see figures and discussions above). Let us now consider the GB dislocations visualized in our HRTEM images, which are responsible for the in-plane rotation. Then, p is perpendicular to ρ . The Frank–Bilby equation can be written as: Here, b is the edge component of the Burgers vectors, ~0.243 nm, and h is the average dislocation spacing. We can then compare the prediction by equation (2) with our experimental observation. From Fig. 3b–e , the measured average dislocation spacing is 0.9, 1.2, 1.6 and 2.0 nm, respectively. The calculated GB angle is correspondingly 15.5°, 11.6°, 8.7° and 7.0°, respectively, which is very consistent with the measured GB angles (15.1°, 11.2°, 8.5° and 7.2°, respectively). From Fig. 4b,c , the measured average dislocation spacing for GB 1–3 is 1.06 and 2.25 nm. The calculated GB angle is then 13.2° and 6.2° for GB 1–3 , also close to the HRTEM measurements of 12.6° and 5.1°. For GB 1–4 , the measured average dislocation spacing is 1.95 and 1.10 nm. The calculated GB angle is 7.1° and 12.7° for GB 1–4 , consistent with the measured GB angle of 7.5° and 15.3° (see summary in Supplementary Table 4 ). It should be noted that for the above application of the Frank–Bilby equation, we only examine the dislocation Burgers vector perpendicular to the tilt GB plane, that is, the edge component of the Burgers vectors, because the screw component of the Burgers vectors cannot be detected and quantified in the HRTEM images. The edge component leads to the rotation, while the screw component (parallel to the GB plane) leads to tilt. In the current study, the mis-orientation angle between grains was defined as the angle between the corresponding lattices of two nearest neighbouring grains observed in the HRTEM imaging. The statistics of the mis-orientation angle distribution of the observed nearest neighbouring grains (that is, 215 nearest neighbouring grain pairs) shows that the GB with mis-orientation angles ranging from 8° to 35° are the high-frequency ones ( Supplementary Fig. 6 ). For high-angle GBs (larger than 15°, per Brandon’s criterion), we also observed collective grain rotation without obvious GB sliding and migration ( Fig. 3 ). This suggests that high-angle GB can also undergo rotation; the mechanism may be similar to that of low-angle GBs, but could also be assisted by possible GB atomic diffusion and shuffling. Cross-grain dislocation-mediated plasticity in larger grains For larger grains, on loading we frequently observed movements and interactions of cross-grain dislocations. 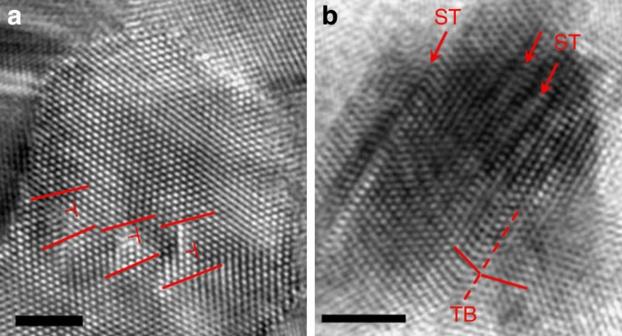Figure 5: HRTEM images show the intra-grain dislocations in larger grains. (a) Full dislocation (marked with ‘T’) in a ~11-nm-sized grain. (b) Partial dislocations resulting in stacking faults (as noted by the arrows) in an ~7-nm-sized grain. Scale bars, 2 nm. Figure 5a provides a typical HRTEM observation of full dislocation (marked with ‘T’) in a ~11-nm-sized grain, with a Burgers vector of a /2[011]. For d between 6 and 10 nm, full dislocations become much less, and stacking faults resulting from the passage of partial dislocations (as noted by the arrows in Fig. 5b ) become more frequent. In fact, >100 grains (with d from 3 to ~25 nm) were monitored during and at the end of the pulling. These include 48 in situ examples, and the others are ex-situ ones (see the many examples in Supplementary Figs 2–11 ). There is a clear trend with decreasing d : the dislocations in action transition from full to partial inside the grains, and eventually to those in the GB to mediate grain rotation. The mechanisms are depicted schematically in Supplementary Fig. 12 . The former (cross-grain dislocation) mechanism has been treated in many previous studies, so our data in that regard are only displayed in Supplementary Materials for interested readers. Figure 5: HRTEM images show the intra-grain dislocations in larger grains. ( a ) Full dislocation (marked with ‘T’) in a ~11-nm-sized grain. ( b ) Partial dislocations resulting in stacking faults (as noted by the arrows) in an ~7-nm-sized grain. Scale bars, 2 nm. Full size image The GB dislocation-mediated grain rotation described here is different from that reported in several earlier experiments on NC metals. In Au with d ~20 nm (ref. 38 ), the grains are sufficiently large that the cross-grain dislocation activities were active and led to the formation of disclinations that move to the GBs. Murayama et al . [39] observed disclination dipoles in bcc Fe and suggested that they may facilitate the re-orientation of grains. Such disclination processes and crystal lattice rotation in the grains are more closely related to grain fragmentation processes [38] , [39] . The grain rotations in these cases are the consequence of cross-grain dislocations [40] , [41] . In recent MD simulations, GB sliding was found to be the controlling mechanism during compressive deformation of Pt [42] . A difference between reference [42] and our observation is that the GBs in their pillar were relaxed within MD timescale only and the specimens were deformed at high strain rates. We now discuss why GB dislocation-mediated grain rotation was observed here, in lieu of GB sliding and diffusional creep. Our experiments were carried out at ~353 K (far below the melting point of Pt, T m =2045 K). At such low temperatures, the GB sliding and diffusional creep only contributed a strain rate well below our experimental strain rate of ~10 −3 s −1 . This is different from the cases of Cu and Au, which have much lower melting temperatures, and the GB sliding and diffusional creep contributions could account for most of the strain rate imposed in experiments. See estimates made in Supplementary Discussion . In comparison, the grain rotation mediated by GB dislocation in Pt can result in a much higher strain rate (of the order of ~3 × 10 −4 s −1 , see Supplementary Discussion ). At d <6 nm, the GB dislocations only need short-distance climb to reach nearby TJs along the GB and climb to free surfaces in the thin film specimens. This explains why GB dislocation-mediated grain rotation becomes favourable when the grain size becomes very small. Our experimental observation of the GB dislocation-controlled grain rotation process involves multiple grains, resembling a grain-switching process in which the coordinates of each individual grain change, as shown in Supplementary Fig. 13 . This is reminiscent of the Ashby–Verrall (A–V) grain-switching model [43] , [44] , [45] . However, in the A–V model, the switching process is through translational movement of an assembly of grains via GB diffusion, rather than rotation via inter-grain dislocation activities only. In the A–V model, the dislocation density along GB does not change dramatically, due to additional help from diffusion and the translational character of the sliding. Our grain rotation is largely of geometry-necessary character with the change in GB dislocation density as the main mechanism, which may be assisted by GB atomic diffusion and shuffling. Although various GB deformation mechanisms have been explored by many groups both experimentally and computationally [11] , [17] , [18] , [21] , [22] , [23] , [24] , [25] , [26] , [46] , [47] , [48] , our results provide for the first time a direct, atomic-scale and quantitative experimental proof that GB dislocation-mediated grain rotation can be active in NC metals near room temperature. Our thin film samples have bottom and top free surfaces and are only a couple of grains thick. A conceivable role of the free surfaces is to enhance atomic diffusion, and dislocation nucleation and climb [49] , [50] , [51] . The very thin films with large free surface areas may have facilitated grain rotation in the current study. For thick samples, grain rotation may still occur via GB dislocations, but may require more accommodation from GB atomic diffusion and shuffling. Recently, the A–V deformation mode was also suggested by MD simulation in both thin films and three-dimensional NC samples [44] , [45] : even when the samples have more than five grains in the thickness direction, grain rotation can still occur via GB dislocations assisted by GB atomic diffusion and shuffling. In conclusion, using in situ atomic scale straining inside TEM, we have captured atomic-scale images of the dynamic processes of grain rotation in Pt nanograins. Our work focuses on a grain size regime ( d <~6 nm) hitherto rarely explored in experiments. In this regime, cross-grain dislocations subside while grain rotation becomes the most prevalent mode. This is a new room-temperature plasticity process in NC metals with extremely small grains, as the grain rotation in this case is found to be mediated by the climb and absorption/generation of Frank–Bilby dislocations in the GB, distinct from the previously proposed mechanism of GB sliding or diffusional creep (e.g., Coble creep). Moreover, our observation has general significance in physical metallurgy, as it directly illustrates for the first time the grain rotation via GB dislocations in a quantitative way consistent with the Frank–Bilby equation. Specifically, the difference in grain orientation (increase or decrease of GB misorientation angle) is entirely accounted for by a change in the density of GB dislocations. In situ TEM tensile device The TEM extensor is made of two thermally actuated bimetallic strips. They were fixed, in opposing positions, on a TEM Cu-ring grid, using superglue or epoxy resin. Each bimetallic strip is made of two layers of different materials (Mn 72 Ni 10 Cu 18 and Fe-Ni 36 alloys) that have a large mismatch in thermal expansion coefficient (26 × 10 −6 and 2.9 × 10 −6 K −1 , respectively), to achieve a significant deflection at relatively low operation temperatures. A significant deflection was clearly visible under gentle heating conditions. The conventional TEM specimen holder (hot stage), now with the bimetallic strips, can therefore act as a double tilt, displacement controlled, deformation stage. The tensile straining of the Pt film was carried out at an estimated strain rate of 10 −3 ~10 −4 . The two bimetallic strips, heated to <80 °C (read from the controller of the sample holder), bent in opposite directions to provide the tensile pulling force. Transferring thin film to the tensile devices A Pt thin film ~10 nm in thickness was deposited on a (001)-oriented NaCl single crystal substrate (3 × 3 cm 2 ) at 300 °C by magnetron sputtering. Operated under optical microscope, the bimetallic extensors (two metallic bars) can be well aligned to be vertical to the thin film samples. Using epoxy resin on the surfaces of the bimetallic extension actuator, the thin films can be attached on the surface of the extensor in almost ideal geometrical configuration. Thus, the uni-axiality of the deformation can be ensured during loading process. Dissolving away the NaCl substrate, free-standing bimetallic strips together with thin film tensile samples are released for loading onto the TEM-tensile stage. During TEM observation, the temperature controller can accurately increase the temperature of the TEM-tensile stage for the bimetallic actuator to exert uniaxial tensile force on the thin films. GB angle measurement method With our double-tilt in situ tensile testing device for TEM, lattice fringe images are easily observed for properly oriented grains. Because of the small scattering angle for electron diffraction, fringe images can be observed for those crystal planes with normal perpendicular to the incident beam direction. The grain rotation (angles) were tracked by grain lattice (fringes) rotation, revealed in HRTEM images. No intra-grain dislocations were revealed in this grain lattice rotation process, and perfect linearity of the grain lattices/fringes were preserved through the grain rotation. It is therefore believed that the rotation is a whole grain rotation. This technique works very well, as long as the axis of rotation is nearly parallel to the electron beam and film normal; otherwise, the lattice fringes will go out of contrast as the diffracting planes are rotated away from the beam. How to cite this article: Wang, L. et al . Grain rotation mediated by grain boundary dislocations in nanocrystalline platinum. Nat. Commun. 5:4402 doi: 10.1038/ncomms5402 (2014).